Identification of a splice variant of mouse TRPA1 that regulates TRPA1 activity Transient receptor potential ankyrin 1 (TRPA1) protein is a nonselective cation channel. Although many studies suggest that TRPA1 is involved in inflammatory and neuropathic pain, its mechanism remains unclear. Here we identify an alternative splice variant of the mouse Trpa1 gene. TRPA1a (full-length) and TRPA1b (splice variant) physically interact with each other and TRPA1b increases the expression of TRPA1a in the plasma membrane. TRPA1a and TRPA1b co-expression significantly increases current density in response to different agonists without affecting their single-channel conductance. Exogenous overexpression of Trpa1b gene in wild-type and TRPA1KO DRG neurons also increases TRPA1a-mediated AITC responses. Moreover, expression levels of Trpa1a and Trpa1b mRNAs change dynamically in two pain models (complete Freund’s adjuvant-induced inflammatory pain and partial sciatic nerve ligation-induced neuropathic pain models). These results suggest that TRPA1 may be regulated through alternative splicing under these pathological conditions. Transient receptor potential (TRP) ion channels are nonselective cation channels that were originally discovered in mutant Drosophila [1] . Many studies revealed that the TRP channel superfamily is important for sensations such as taste, pain and temperature, both in the peripheral and central nervous systems [2] , [3] . The TRP channel superfamily is now divided into seven subfamilies: TRPV (Vanilloid), TRPC (Canonical), TRPM (Melastatin), TRPML (Mucolipin), TRPN (NompC), TRPP (Polycystic) and TRPA (Ankyrin). TRPA1 is the only member of the TRPA subfamily in mammals, with the presence of up to 17 ankyrin repeat domains [4] . TRPA1 channel is predominantly expressed in sensory neurons [3] , while there is some expression in other cell types such as astrocytes, enterochromaffin cells and pancreatic β-cells [5] , [6] , [7] . In sensory neurons of the dorsal root ganglion (DRG) and trigeminal ganglion (TG), TRPA1 channels are predominately expressed in small-diameter neurons. They are believed to be involved in many forms of nociception, with some reports suggesting that nerve growth factor regulates chronic inflammatory hyperalgesia by controlling Trpa1 gene expression [8] . Alternative splicing of pre-mRNA was identified more than 30 years ago when it was discovered that two proteins could be encoded by the same gene [9] , [10] . Alternative splicing is a complex regulatory mechanism in eukaryotes by which protein diversity is increased from a relatively small number of genes [11] . More than 95% of human genes are estimated to undergo alternative splicing [12] , [13] . Alternative splicing also has an important role during cell differentiation and development in a time- and tissue-specific manner [14] , [15] . Recently, two studies identified several alternative splice variants of TrpA1 in Drosophila that were expressed in a tissue-specific manner and displayed different chemical and thermal sensitivities [16] , [17] . However, to date, there has been no reports of a mammalian TRPA1 splice variant, even though there are some instances of other TRP channels undergoing alternative splicing [18] , [19] . For instance, an alternative splice variant of Trpv1 was reported to be a dominant-negative isoform [20] . In this study, a splice variant of the mouse Trpa1 gene is identified and cloned from DRG neurons. This splice variant skips exon 20, which encodes 30 amino acids. The full-length TRPA1 protein is designated TRPA1a and the splice variant as TRPA1b. TRPA1a and TRPA1b physically interact with each other. Co-expression of TRPA1a with TRPA1b significantly increases TRPA1 agonist responses. Moreover, dynamic changes in Trpa1a and Trpa1b expression levels are observed under inflammatory and neuropathic pain conditions. These results suggest TRPA1 might be involved in these pathologic conditions through alternative splicing. Cloning a mouse Trpa1 alternative splice variant TRPA1 is predominantly expressed in DRG and TG neurons and functions as a nociceptive receptor [3] , [21] . Starting with RNA from mouse DRG neurons, RT–PCR analysis revealed an additional fragment using primers designed to amplify a partial fragment of mouse Trpa1 mRNA ( Fig. 1a ), suggesting that this additional fragment was an alternative splice variant. To confirm that this result was not due to non-specific amplification, two fragments were extracted from the agarose gel and sequenced. The additional fragment indeed corresponded to a Trpa1 splice variant whose sequence was confirmed by rapid amplification of cDNA ends using RNA from mouse DRG neurons. The splice variant excluded exon 20, which contained 90 bp. Full-length mRNA was referred to as Trpa1a and the variant as Trpa1b ( Fig. 1b ). The amino-acid sequence of the TRPA1a protein is identical to the previously reported TRPA1 channel that contains 1,125 amino acids [3] . As there was no reading frame shifting, TRPA1b excluded only the sequence corresponding to the 30 amino acids from 777 to 807 in TRPA1a, resulting in a protein of 1,095 amino acids. The deleted amino acids were in the second transmembrane domain and the first intracellular loop ( Fig. 1c ). Trpa1a and Trpa1b mRNAs were expressed in DRG and TG as well as in small intestine and colon, although both Trpa1a and Trpa1b expression in small intestine and colon was relatively weaker than that in DRG and TG ( Fig. 1d ). Single-cell RT–PCR analysis confirmed that Trpa1a and Trpa1b were expressed in the same DRG neurons together with Trpv1 ( Fig. 1e ). Although the nucleotide sequence of exon 20 is highly conserved among mouse, and rat Trpa1 and human TRPA1 ( Supplementary Fig. S1a ), no additional RT–PCR fragment was amplified using rat and human RNAs, indicating that this splice variant could be mouse-specific ( Supplementary Fig. S1b ). Using DRG samples collected from 10 mice, two protein bands were successfully detected ( Fig. 1f , right panel). They corresponded to the sizes of TRPA1a and TRPA1b expressed in HEK293T cells ( Fig. 1f , left panel and Supplementary Fig. S2 ). These two bands were not affected by treatment with a deglycosylation enzyme for 4 hours, indicating that these proteins were not glycosylated and non-glycosylated forms of TRPA1, respectively ( Supplementary Fig. S3 ). 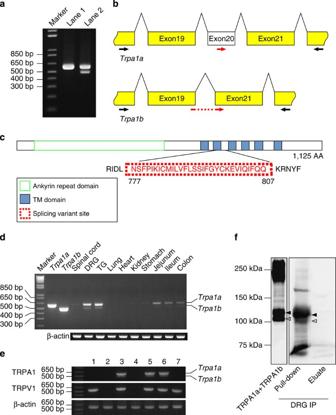Figure 1: Identification of an alternative splice variant of the mouseTrpa1gene from DRG cells. (a) Representative results for RT–PCR using mouse DRG. Lane 1:Trpa1a-positive control; Lane 2: cDNA from mouse DRG. (b) SchematicTrpa1aandTrpa1bmRNA structures. Black arrows indicate the forward and reverse primers for RT–PCR analysis and red arrows indicate forward primers for qRT–PCR analysis. (c) Schematic protein structure of the TRPA1 channel. The dot red box indicates the 30 amino acid residues missing in the TRPA1b protein. The green box indicates the ankyrin repeat domain and the six blue boxes indicate the six predicted transmembrane domains of TRPA1a. (d) Specific expression patterns ofTrpa1aandTrpa1bmRNAs were confirmed by RT–PCR analysis of different mouse tissues. (e) Single-cell RT–PCR from mouse DRG neurons. Numbers indicate PCR results from different neurons. Expected sizes of the amplified fragments are 577 bp, 548 bp and 573 bp forTrpa1,Trpv1and β-actin, respectively. (f) Western blotting result after immunoprecipitation of TRPA1 from mouse DRG with an anti-mouse TRPA1 antibody. Black and white arrowheads indicate TRPA1a and TRPA1b proteins, respectively. Figure 1: Identification of an alternative splice variant of the mouse Trpa1 gene from DRG cells. ( a ) Representative results for RT–PCR using mouse DRG. Lane 1: Trpa1a -positive control; Lane 2: cDNA from mouse DRG. ( b ) Schematic Trpa1a and Trpa1b mRNA structures. Black arrows indicate the forward and reverse primers for RT–PCR analysis and red arrows indicate forward primers for qRT–PCR analysis. ( c ) Schematic protein structure of the TRPA1 channel. The dot red box indicates the 30 amino acid residues missing in the TRPA1b protein. The green box indicates the ankyrin repeat domain and the six blue boxes indicate the six predicted transmembrane domains of TRPA1a. ( d ) Specific expression patterns of Trpa1a and Trpa1b mRNAs were confirmed by RT–PCR analysis of different mouse tissues. ( e ) Single-cell RT–PCR from mouse DRG neurons. Numbers indicate PCR results from different neurons. Expected sizes of the amplified fragments are 577 bp, 548 bp and 573 bp for Trpa1 , Trpv1 and β-actin, respectively. ( f ) Western blotting result after immunoprecipitation of TRPA1 from mouse DRG with an anti-mouse TRPA1 antibody. Black and white arrowheads indicate TRPA1a and TRPA1b proteins, respectively. Full size image Physical interaction between TRPA1a and TRPA1b As TRPA1a and TRPA1b differed by only 30 amino acid residues, there was no antibody available that could efficiently differentiate between them. Therefore, tagged constructs of TRPA1a-EGFP and TRPA1b-FLAG were generated for further analysis. After heterologous expression in HEK293T cells, TRPA1a-EGFP and TRPA1b-FLAG signals were detected using EGFP fluorescence (green) and an anti-FLAG antibody (red), respectively ( Fig. 2a ). HEK293T cells co-expressing TRPA1a-EGFP with TRPA1b-FLAG displayed essentially similar EGFP fluorescence and FLAG immunoreactivity compared with cells expressing either TRPA1a-EGFP or TRPA1b-FLAG alone. In addition, TRPA1a-EGFP and TRPA1b-FLAG were highly colocalized on the plasma membrane of HEK293T cells co-expressing the two proteins together ( Fig. 2a , Merged). As both TRPA1a and TRPA1b were expressed in the same neurons, it was possible that they physically interacted with each other. This possibility was confirmed by co-immunoprecipitation experiments in that there was indeed a physical interaction between TRPA1a and TRPA1b when they were heterologously expressed in HEK293T cells ( Fig. 2b ). Interestingly, in the native-PAGE analysis, HEK293T cells co-expressing TRPA1a-EGFP with TRPA1b-FLAG showed a larger size band ( Fig. 2c , white arrowheads, ~920 kDa) compared with cells expressing TRPA1a-EGFP homo-tetramer ( Fig. 2c , red arrowhead, ~600 kDa) or TRPA1b-FLAG homo-tetramer ( Fig. 2c , black arrowhead, ~520 kDa). The native-PAGE result further supported the idea that TRPA1a and TRPA1b physically interacted with each other and formed a large complex. 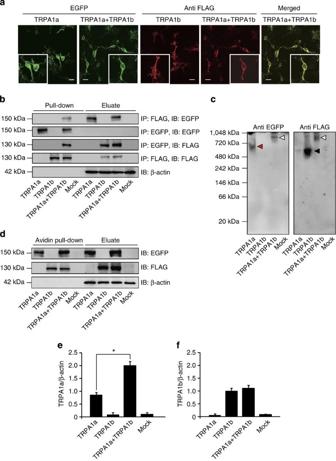Figure 2: TRPA1b physically interacts with TRPA1a and regulates its plasma membrane expression. (a) Immunocytochemical analysis of TRPA1a and TRPA1b protein expression in HEK293T cells using TRPA1a-EGFP and TRPA1b-FLAG proteins. Green colour images indicate the cells were stimulated with EGFP fluorescence, whereas red colour images indicate the cells were stained with an anti-FLAG antibody. A merged image (yellow) shows the expression of both TRPA1a-EGFP and TRPA1b-FLAG. Small square boxes indicate the magnified images. Scale bars indicate 20 μm. (b) Co-immunoprecipitation results of TRPA1a-EGFP and/or TRPA1b-FLAG protein expression in HEK293T cells. Proteins were immunoprecipitated and immunoblotted with either anti-EGFP or anti-FLAG antibody. β-actin was the loading control for all of the groups. (c) The native-PAGE analysis for TRPA1a-EGFP and TRPA1b-FLAG using an anti-EGFP or anti-FLAG antibody, respectively. Red and black arrowheads possibly indicate TRPA1a and TRPA1b homo-tetramers, respectively. White arrowheads possibly indicate the complex formed by TRPA1a and TRPA1b. (d) Immunoblotting analysis of TRPA1a and TRPA1b protein expression in biotin-labeled plasma membranes. (e,f) Quantitative analysis of the expression of TRPA1a (e) and TRPA1b (f) proteins in the plasma membrane relative to β-actin. Data represent mean±s.e.m. *P<0.05,n=5, one-way ANOVA with Bonferroni’spost hocanalysis. Figure 2: TRPA1b physically interacts with TRPA1a and regulates its plasma membrane expression. ( a ) Immunocytochemical analysis of TRPA1a and TRPA1b protein expression in HEK293T cells using TRPA1a-EGFP and TRPA1b-FLAG proteins. Green colour images indicate the cells were stimulated with EGFP fluorescence, whereas red colour images indicate the cells were stained with an anti-FLAG antibody. A merged image (yellow) shows the expression of both TRPA1a-EGFP and TRPA1b-FLAG. Small square boxes indicate the magnified images. Scale bars indicate 20 μm. ( b ) Co-immunoprecipitation results of TRPA1a-EGFP and/or TRPA1b-FLAG protein expression in HEK293T cells. Proteins were immunoprecipitated and immunoblotted with either anti-EGFP or anti-FLAG antibody. β-actin was the loading control for all of the groups. ( c ) The native-PAGE analysis for TRPA1a-EGFP and TRPA1b-FLAG using an anti-EGFP or anti-FLAG antibody, respectively. Red and black arrowheads possibly indicate TRPA1a and TRPA1b homo-tetramers, respectively. White arrowheads possibly indicate the complex formed by TRPA1a and TRPA1b. ( d ) Immunoblotting analysis of TRPA1a and TRPA1b protein expression in biotin-labeled plasma membranes. ( e , f ) Quantitative analysis of the expression of TRPA1a ( e ) and TRPA1b ( f ) proteins in the plasma membrane relative to β-actin. Data represent mean±s.e.m. * P <0.05, n =5, one-way ANOVA with Bonferroni’s post hoc analysis. Full size image Plasma membrane localization is important for TRPA1 channel function. Thus, interaction between TRPA1a and TRPA1b could affect their plasma membrane expression levels. To examine this possibility, a biotinylation assay of plasma membrane proteins was performed. After biotin labelling, plasma membrane proteins were pulled down with avidin-beads and immunoreacted with the appropriate primary antibodies. Both TRPA1a and TRPA1b were confirmed to translocate to the plasma membrane ( Fig. 2d ), with TRPA1a plasma membrane levels significantly increased upon co-expression with TRPA1b compared with cells expressing TRPA1a alone ( Fig. 2e ). The plasma membrane expression level of TRPA1b was not changed ( Fig. 2f ). These results indicated that TRPA1a and TRPA1b physically interacted with each other and that co-expression of TRPA1a with TRPA1b enhanced TRPA1a expression on the plasma membrane. TRPA1a and TRPA1b co-expression influences TRPA1 activity The increased TRPA1 protein expression observed above could lead to enhanced TRPA1 activity. To examine this possibility, electrophysiological experiments using both TRPA1a and TRPA1b were performed using a whole-cell patch-clamp method. Mock-transfected HEK293T cells were confirmed not to respond to 100 μM allyl isothiocyanate (AITC), whereas cells expressing TRPA1a showed a large inward current. Unexpectedly, cells expressing TRPA1b alone failed to respond to AITC; however, HEK293T cells co-expressing TRPA1a with TRPA1b exhibited a larger inward current than that of cells expressing TRPA1a alone. The outward-rectifying current–voltage relationships were similar in cells expressing TRPA1a alone and cells expressing TRPA1a with TRPA1b ( Fig. 3a ). 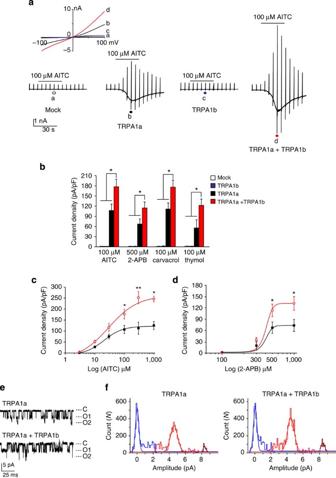Figure 3: Co-expression of TRPA1b increases TRPA1a current density in HEK293T cells. (a) Representative whole-cell current traces and current-voltage (I–V) relationship curves in response to 100 μM AITC in control (Mock) cells and cells expressing TRPA1a alone, TRPA1b alone or TRPA1a with TRPA1b. a, b, c, and d in the traces indicate the point at whichI–Vcurves were generated. (b) Comparison of TRPA1-mediated current densities activated by four different agonists. Data represent mean±s.e.m. *P<0.05,n≥11 each, one-way ANOVA with Bonferroni’spost hocanalysis. (c,d) Dose-dependent curves for AITC-evoked (c) and 2-APB-evoked (d) responses. Red open circles indicate responses in HEK293T cells expressing both TRPA1a and TRPA1b, and black squares indicate responses in cells expressing TRPA1a alone. Data represent mean±s.e.m. *P<0.05; **P<0.01,n≥8 and 9, respectively, unpaired Student’st-test. (e) Representative 100 μM AITC-evoked single-channel current traces from cells expressing TRPA1a alone (upper) and cells expressing TRPA1a and TRPA1b (lower). Holding potential is −60 mV. (f) Open-event histograms of 100 μM AITC-evoked single-channel responses from cells expressing TRPA1a alone (left) and cells expressing TRPA1a and TRPA1b (right). Average single-channel conductance was 60.8±2.6 pS for cells expressing TRPA1a alone and 63.3±3.0 pS for cells expressing TRPA1a with TRPA1b. TRPA1an=20; TRPA1a+TRPA1bn=23. Figure 3: Co-expression of TRPA1b increases TRPA1a current density in HEK293T cells. ( a ) Representative whole-cell current traces and current-voltage ( I – V ) relationship curves in response to 100 μM AITC in control (Mock) cells and cells expressing TRPA1a alone, TRPA1b alone or TRPA1a with TRPA1b. a, b, c, and d in the traces indicate the point at which I – V curves were generated. ( b ) Comparison of TRPA1-mediated current densities activated by four different agonists. Data represent mean±s.e.m. * P <0.05, n ≥11 each, one-way ANOVA with Bonferroni’s post hoc analysis. ( c , d ) Dose-dependent curves for AITC-evoked ( c ) and 2-APB-evoked ( d ) responses. Red open circles indicate responses in HEK293T cells expressing both TRPA1a and TRPA1b, and black squares indicate responses in cells expressing TRPA1a alone. Data represent mean±s.e.m. * P <0.05; ** P <0.01, n ≥8 and 9, respectively, unpaired Student’s t -test. ( e ) Representative 100 μM AITC-evoked single-channel current traces from cells expressing TRPA1a alone (upper) and cells expressing TRPA1a and TRPA1b (lower). Holding potential is −60 mV. ( f ) Open-event histograms of 100 μM AITC-evoked single-channel responses from cells expressing TRPA1a alone (left) and cells expressing TRPA1a and TRPA1b (right). Average single-channel conductance was 60.8±2.6 pS for cells expressing TRPA1a alone and 63.3±3.0 pS for cells expressing TRPA1a with TRPA1b. TRPA1a n =20; TRPA1a+TRPA1b n =23. Full size image AITC activates TRPA1 through covalent modification of cysteine residues [22] , [23] , but TRPA1 can also be activated by different compounds that do not promote covalent modification [24] , [25] , [26] . Three other TRPA1 agonists (2-APB, carvacrol and thymol) that are known to activate TRPA1 through non-covalent modification mechanisms were used [27] . As with AITC, none of these agonists induced inward current in HEK293T cells expressing TRPA1b alone, whereas they all induced significantly larger inward currents in HEK293T cells co-expressing TRPA1a with TRPA1b compared with cells expressing TRPA1a alone ( Fig. 3b ). These results strongly suggested that, regardless of the activation mechanisms, co-expression of TRPA1a with TRPA1b caused significantly larger agonist-induced TRPA1 currents compared with cells expressing TRPA1a alone. These significantly increased currents could be easily explained by the biotinylation assay results that showed an increased plasma membrane expression level of TRPA1a upon co-expression with TRPA1b in HEK293T cells ( Fig. 2 ). As TRPA1 was initially reported as a sensor for noxious cold stimulus [3] , cold response was also examined. However, neither TRPA1a, TRPA1b nor TRPA1a+TRPA1b was activated by cold stimulus (as low as 10 °C) in the absence or presence of 100 nM intracellular calcium, supposedly an enhancer of TRPA1 activity [28] ( Supplementary Fig. S4 ). These results indicated that TRPA1a with or without TRPA1b was cold-insensitive. In addition, different transfection ratios of TRPA1a and TRPA1b were examined. Even co-expression of TRPA1a with TRPA1b at a ratio of 2:1 significantly enhanced the current density in response to 300 μM AITC, and the enhancement was saturated with a ratio of 1:1. This result indicated that TRPA1b interacted with TRPA1a in a concentration-dependent manner ( Supplementary Fig. S5 ). To clarify whether co-expression of TRPA1a with TRPA1b influenced the activation properties of TRPA1a, the effects of different concentrations of agonists, AITC and 2-APB on TRPA1-mediated currents were examined and dose-dependent curves for AITC- and 2-APB-evoked responses were fitted to Hill equations ( Fig. 3c,d ). The calculated EC 50 values for AITC- and 2-APB-induced activation ( Table 1 ) were quite similar to those stated in a previous report [29] . Although co-expression of TRPA1a with TRPA1b did not affect the Hill coefficients or the EC 50 values of these two curves compared with TRPA1a expression alone, the maximum current density (CD max ) in response to both AITC and 2-APB was significantly larger in cells co-expressing TRPA1a with TRPA1b compared with cells expressing TRPA1a alone ( Table 1 and Fig. 3c,d ). These results suggested that co-expression of TRPA1a with TRPA1b increased the efficacy but not the potency of AITC and 2-APB actions on TRPA1. This observation was consistent with the two-fold increase in the plasma membrane expression level of TRPA1a upon co-expression with TRPA1b ( Fig. 2e ). Table 1 Parameters of AITC and 2-APB-activated TRPA1 responses in TRP-expressing HEK293T cells. Full size table If TRPA1a and TRPA1b physically interacted with each other by forming a heteromer, the single-channel properties could be affected. To examine this possibility, inside-out single-channel recordings were performed in HEK293T cells expressing TRPA1a alone and in cells co-expressing TRPA1a with TRPA1b ( Fig. 3e ). Surprisingly, TRPA1a and TRPA1b co-expression did not affect open-time kinetics ( Supplementary Fig. S6 ) or single-channel conductance ( Table 2 ). However, NP o values from cells expressing TRPA1a with TRPA1b in response to 100 μM AITC were significantly higher than those from cells expressing TRPA1a alone ( Fig. 3f and Table 2 ). These results could be explained by an increase in channel number in the patch membrane. These data suggested that the increase in agonist responses was possibly due to the enhanced expression levels of TRPA1a by co-expression with TRPA1b, but not changing the single-channel conductance. Table 2 Single-channel recordings from TRP-expressing HEK293T cells. Full size table TRPA1b interacts and regulates TRPA1a in DRG neurons All studies thus far had been performed using a heterologous expression system with HEK293T cells. Next, mouse DRG neurons were chosen to confirm the TRPA1a and TRPA1b interaction observed in HEK293T cells. Trpa1b gene was overexpressed in WT DRG neurons by electroporation. WT DRG neurons treated with vector pcDNA3.1 served as Control. The changes in fura-2 ratio corresponding to cytosolic calcium concentrations ([Ca 2+ ] i ) of the DRG neurons were recorded in response to AITC (100 μM) and capsaicin (Cap, 0.5 μM) ( Fig. 4a ). The responses were normalized to those of ionomycin and statistically analysed. The data indicated that AITC-, but not Cap-evoked ratio increases were significantly larger in TRPA1b-overexpressing neurons compared with that in control neurons ( Fig. 4b ). As previous reports showed that DRG neurons have distinct TRP channel expression patterns [2] , [8] , [30] , cell populations were also compared between Control and TRPA1b overexpressing DRG neurons. Overexpression of TRPA1b did not significantly influence endogenous TRP channel expression patterns ( Fig. 4c ), indicating that TRPA1b only affected TRPA1a but not the TRPV1 channel. In addition, changes in real [Ca 2+ ] i in response to AITC were calculated from these two groups using a standard curve. The results showed that mouse DRG neurons expressing exogenous TRPA1b had a significantly larger increase in [Ca 2+ ] i ( Supplementary Fig. S7 ), similar to the results calculated from the normalized ratio. 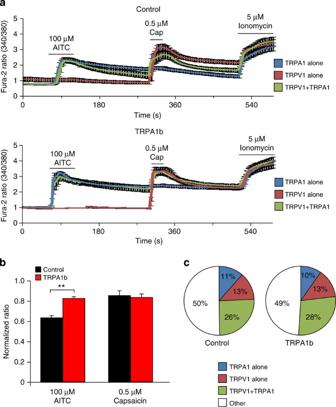Figure 4: TRPA1b overexpression in WT DRG cells enhanced the AITC- but not the capsaicin-evoked increase in the fura-2 ratio. (a) Changes in the fura-2 ratio in vector-introduced (Control, upper) and TRPA1b-introduced (lower) DRG neurons from WT mice. Black bars indicate agonist application periods. Responses to TRPA1 alone (blue), TRPV1 alone (red), and TRPA1 with TRPV1 (green) are shown. (b) AITC and Cap responses (normalized to the ionomycin responses) were compared. Data represent mean±s.e.m. **P<0.01, Controln=343; TRPA1bn=308, unpaired Student’st-test. (c) Summary of AITC- and Cap-positive cell populations from vector-introduced (Control, left) and TRPA1b-introduced (right) DRG neurons. Figure 4: TRPA1b overexpression in WT DRG cells enhanced the AITC- but not the capsaicin-evoked increase in the fura-2 ratio. ( a ) Changes in the fura-2 ratio in vector-introduced (Control, upper) and TRPA1b-introduced (lower) DRG neurons from WT mice. Black bars indicate agonist application periods. Responses to TRPA1 alone (blue), TRPV1 alone (red), and TRPA1 with TRPV1 (green) are shown. ( b ) AITC and Cap responses (normalized to the ionomycin responses) were compared. Data represent mean±s.e.m. ** P <0.01, Control n =343; TRPA1b n =308, unpaired Student’s t -test. ( c ) Summary of AITC- and Cap-positive cell populations from vector-introduced (Control, left) and TRPA1b-introduced (right) DRG neurons. Full size image TRPA1KO DRG neurons were also used to further examine the effects of TRPA1a and TRPA1b. TRPA1KO DRG neurons were electroporated with either control (pcDNA3.1), TRPA1a alone or TRPA1a with TRPA1b plasmid DNAs. Expression of TRPA1a alone and TRPA1a with TRPA1b rescued responses to AITC in the TRPA1KO neurons, whereas control cells showed no response ( Fig. 5a ). Interestingly, we observed a significantly larger ratio change in neurons co-expressing TRPA1a with TRPA1b compared with those expressing TRPA1a alone ( Fig. 5b ), similar to the experiment performed with WT neurons ( Fig. 4b and Supplementary Fig. S7 ). Taken together, these results suggested that TRPA1b not only regulated TRPA1a expression in the heterologous expression system with HEK293T cells but also regulated TRPA1a expression in native sensory neurons. 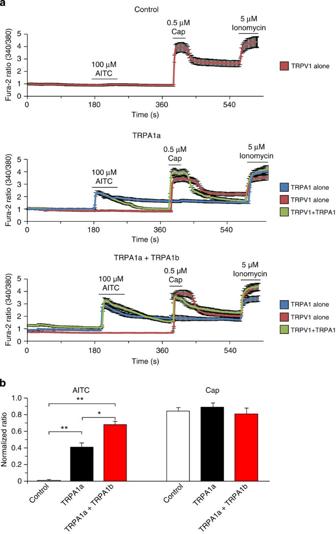Figure 5: Exogenous expression of TRPA1a and TRPA1b rescued the AITC-evoked increase in the fura-2 ratio in TRPA1KO DRG cells. (a) Changes in the fura-2 ratio in vector-introduced (Control, upper), TRPA1a-introduced (middle) and TRPA1a with TRPA1b-introduced (lower) DRG neurons from TRPA1KO mice. Black bars indicate agonist application periods. Responses to TRPA1 alone (blue), TRPV1 alone (red) and TRPV1 with TRPA1 (green) are shown. (b) AITC responses (normalized to the ionomycin responses) were compared. Data represent mean±s.e.m. *P<0.05, **P<0.01, Controln=298; TRPA1an=312; TRPA1a+TRPA1bn=298, one-way ANOVA with Bonferroni’spost hocanalysis. Figure 5: Exogenous expression of TRPA1a and TRPA1b rescued the AITC-evoked increase in the fura-2 ratio in TRPA1KO DRG cells. ( a ) Changes in the fura-2 ratio in vector-introduced (Control, upper), TRPA1a-introduced (middle) and TRPA1a with TRPA1b-introduced (lower) DRG neurons from TRPA1KO mice. Black bars indicate agonist application periods. Responses to TRPA1 alone (blue), TRPV1 alone (red) and TRPV1 with TRPA1 (green) are shown. ( b ) AITC responses (normalized to the ionomycin responses) were compared. Data represent mean±s.e.m. * P <0.05, ** P <0.01, Control n =298; TRPA1a n =312; TRPA1a+TRPA1b n =298, one-way ANOVA with Bonferroni’s post hoc analysis. Full size image Changes of Trpa1a and Trpa1b mRNAs in two animal models Recent studies suggested that activation of TRPA1 contributes to mechanical hyperalgesia under inflammatory pain conditions [31] , [32] , where Trpa1 mRNA was found to increase rapidly and then return to basal level [8] , [33] . However, the regulatory mechanism of TRPA1 involvement in inflammatory pain conditions has remained unclear. Therefore, a complete Freund’s adjuvant (CFA)-induced inflammatory pain model was used to explore whether TRPA1b modulated TRPA1a under pathological pain conditions. In WT mice, intraplantar injection of CFA into the hind paw induced mechanical hyperalgesia that was confirmed by the von Frey filament test. The reduction lasted for 14 days and was not observed in the control mice injected with saline. Intraplantar injection of CFA into TRPA1KO mice hind paws, however, significantly reduced the ipsilateral 50% mechanical threshold only on days 1 and 2 ( Fig. 6a ). These findings indicate that TRPA1 function is of greater importance in the later stage of inflammation. No significant changes in the 50% mechanical threshold of the contralateral hind paws were observed among the three groups tested ( Supplementary Fig. S8a ). The expression levels of Trpa1 mRNA in mouse DRG neurons from lumbar 4, 5 and 6 sections, which correspond to the affected hind paw neurons, were evaluated by qRT–PCR analysis at different time points after the injection. The expression level of Trpa1a mRNA from ipsilateral DRG neurons of CFA-injected mice was significantly increased on day 1 compared with that from ipsilateral DRG neurons of saline-injected mice ( Fig. 6c ). The increased Trpa1a expression level returned to basal level on day 5 after injection, which is consistent with the previous studies [8] , [33] . On the other hand, the expression level of Trpa1b mRNA gradually but significantly increased for 14 days after injection ( Fig. 6d ). No significant difference was observed in either Trpa1a or Trpa1b mRNA expression level from contralateral DRG cells of these groups ( Supplementary Fig. S8c ). Functional analysis of TRPA1 was examined by using a calcium-imaging method ( Fig. 6g ). Consistent with the behavioural results, AITC responses in ipsilateral DRG neurons from CFA-injected WT mice were significantly larger compared with those in DRG neurons from saline-injected WT mice. DRG neurons from TRPA1KO mice did not respond to AITC. Furthermore, contralateral DRG neurons did not exhibit significant differences in AITC responses between saline- and CFA-injected mice ( Supplementary Fig. S8e ). 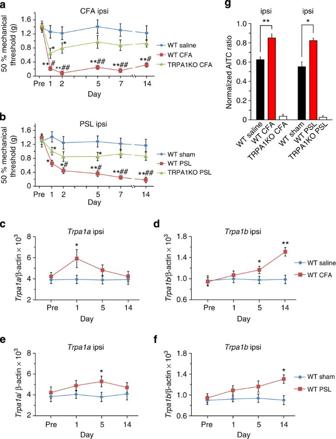Figure 6: Behavioural analysis and mRNA expression patterns ofTrpa1aandTrpa1bin two pain models. (a,b) Changes in the ipsilateral 50% mechanical thresholds of CFA-induced inflammatory pain (a) and PSL-induced neuropathic pain (b) models. Data represent mean±s.e.m. *P<0.05, **P<0.01 versus WT saline or sham, #P<0.05, ##P<0.01 versus TRPA1KO CFA or PSL, WT saline (blue)n=36; WT CFA (red)n=48; TRPA1KO CFA (green)n=5; WT sham (blue)n=40; WT PSL (red)n=44; TRPA1KO PSL (green)n=5, one-way ANOVA with Bonferroni’spost hocanalysis. (c,d) Time courses ofTrpa1a(c) andTrpa1b(d) mRNA expression levels in ipsilateral DRG from CFA-induced inflammatory pain model. Data represent mean±s.e.m. *P<0.05, **P<0.01 versus WT saline, WT salinen=9; WT CFAn=12, unpaired Student’st-test. (e,f) Time courses ofTrpa1a(e) andTrpa1b(f) mRNA expression levels in ipsilateral DRG from PSL-induced neuropathic pain model. Data represent mean±s.e.m. *P<0.05, **P<0.01 versus WT sham, WT shamn=10; WT PSLn=11, unpaired Student’st-test. (g) Changes in the fura-2 ratio in ipsilateral DRG 2 weeks after CFA-injection and PSL-operation. Saline-injected and sham-operated WT mice (black), CFA-injected and PSL-operated WT mice (red), CFA-injected and PSL-operated TRPA1KO mice (white). Data represent mean±s.e.m. *P<0.05, **P<0.01 versus WT saline or sham, WT salinen=275; WT CFAn=286; TRPA1KO CFAn=284; WT shamn=239; WT PSLn=275; TRPA1KO PSLn=300, one-way ANOVA with Bonferroni’spost hocanalysis. Figure 6: Behavioural analysis and mRNA expression patterns of Trpa1a and Trpa1b in two pain models. ( a , b ) Changes in the ipsilateral 50% mechanical thresholds of CFA-induced inflammatory pain ( a ) and PSL-induced neuropathic pain ( b ) models. Data represent mean±s.e.m. * P <0.05, ** P <0.01 versus WT saline or sham, # P <0.05, ## P <0.01 versus TRPA1KO CFA or PSL, WT saline (blue) n =36; WT CFA (red) n =48; TRPA1KO CFA (green) n =5; WT sham (blue) n =40; WT PSL (red) n =44; TRPA1KO PSL (green) n =5, one-way ANOVA with Bonferroni’s post hoc analysis. ( c , d ) Time courses of Trpa1a ( c ) and Trpa1b ( d ) mRNA expression levels in ipsilateral DRG from CFA-induced inflammatory pain model. Data represent mean±s.e.m. * P <0.05, ** P <0.01 versus WT saline, WT saline n =9; WT CFA n =12, unpaired Student’s t -test. ( e , f ) Time courses of Trpa1a ( e ) and Trpa1b ( f ) mRNA expression levels in ipsilateral DRG from PSL-induced neuropathic pain model. Data represent mean±s.e.m. * P <0.05, ** P <0.01 versus WT sham, WT sham n =10; WT PSL n =11, unpaired Student’s t -test. ( g ) Changes in the fura-2 ratio in ipsilateral DRG 2 weeks after CFA-injection and PSL-operation. Saline-injected and sham-operated WT mice (black), CFA-injected and PSL-operated WT mice (red), CFA-injected and PSL-operated TRPA1KO mice (white). Data represent mean±s.e.m. * P <0.05, ** P <0.01 versus WT saline or sham, WT saline n =275; WT CFA n =286; TRPA1KO CFA n =284; WT sham n =239; WT PSL n =275; TRPA1KO PSL n =300, one-way ANOVA with Bonferroni’s post hoc analysis. Full size image Some research has demonstrated that TRPA1 has an important role in neuropathic pain [8] , [34] , [35] , [36] , whereas other studies did not support that conclusion [37] , [38] , [39] . In this study, a partial sciatic nerve ligation (PSL)-induced neuropathic pain model was selected to examine the involvement of TRPA1 and to determine the mRNA expression levels of Trpa1a and Trpa1b . The same experimental time course paradigm was applied to WT sham-operated, WT PSL-operated and TRPA1KO PSL-operated mice as in the CFA-induced inflammatory pain model. The 50% mechanical threshold was significantly reduced in PSL-operated WT mice 1 day after ligation compared with sham-operated WT mice. The reduced mechanical threshold gradually reached a plateau on day 14 after ligation. Interestingly, PSL-operated TRPA1KO mice exhibited only a partial reduction in the 50% mechanical threshold ( Fig. 6b ), which suggested that TRPA1 could be involved in PSL-induced mechanical hypersensitivity to some extent. No significant changes in the 50% mechanical threshold of the contralateral hind paws were observed in the three groups tested ( Supplementary Fig. S8b ). In ipsilateral DRG from PSL-operated WT mice, the Trpa1a mRNA expression level significantly increased on day 5 after ligation and returned to the basal level on day 14 ( Fig. 6e ). On the other hand, the Trpa1b mRNA expression level gradually increased for 14 days after ligation ( Fig. 6f ). However, neither the Trpa1a nor Trpa1b mRNA expression level was significantly changed in contralateral DRG neurons in PSL-operated or sham-operated mice ( Supplementary Fig. S8d ). Similar to the results obtained with the CFA model, AITC responses in ipsilateral DRG neurons from PSL-operated WT mice were significantly larger compared with those in DRG neurons from sham-operated WT mice ( Fig. 6g ). DRG neurons from TRPA1KO mice did not respond to AITC. In addition, contralateral DRG did not exhibit significant differences in AITC responses between sham- and PSL-operated mice ( Supplementary Fig. S8e ). Therefore, the mRNA expression levels and functional analysis results indicated that TRPA1a is involved in both pain models (CFA-induced inflammatory pain and PSL-induced neuropathic pain models). These data indicate that TRPA1a could be regulated by its alternative splice variant TRPA1b in the late stages of these conditions. TRPA1 is reportedly expressed in a subpopulation of peptidergic sensory neurons that also co-express TRPV1 (ref. 3 ). It can be activated in response to many chemicals, natural plant extracts and a large number of pro-algesic agents [40] , [41] . Activation of TRPA1 in sensory neurons causes pain-related behaviours in mice [3] , whereas TRPA1KO mice are insensitive to TRPA1 agonists and display impaired pain-related behaviours in response to these compounds [21] . TRPA1KO mice also did not develop neurogenic inflammation and hyperalgesia compared with WT animals [34] , [42] . These results suggest that TRPA1 is not only the primary receptor for these compounds in nociceptive neurons but also is involved in inflammatory and neuropathic pain diseases where mechanical hyperalgesia is observed. However, the mechanisms for the latter phenomena are not completely understood. In the present study, we identified a mouse-specific alternative splice isoform of the TRPA1 channel, TRPA1b, which lost part of TM2 and the adjacent intracellular loop. The loss of these 30 amino acids would seem likely to create a non-functional channel. This would explain why TRPA1b alone has no activity and would also be consistent with TRPA1b having no effect on the single-channel properties of TRPA1a currents. These results might suggest that TRPA1b functions as a dominant-negative isoform. However, it was not the case, and instead TRPA1b seems to make TRPA1a more active or at least more prevalent on the cell surface. Moreover, we observed that dynamic changes in mRNA expression levels of Trpa1a and Trpa1b occurred under inflammatory and neuropathic pain conditions. Trpa1a and Trpa1b mRNAs were found to co-exist in the same DRG neurons. Co-immunoprecipitation confirmed that TRPA1a and TRPA1b physically interacted with each other. Interestingly, the membrane expression level of TRPA1a significantly increased upon co-expression with TRPA1b. Although the detailed mechanism remains unclear, it is possible that translocation of TRPA1a could be enhanced by physical interaction with TRPA1b. Alternatively, it is possible that the stability or rate of internalization of the complex could be affected by TRPA1b, which would be analogous to the findings of several studies showing that splice variants have different internalization or post-endocytic sorting fates [43] , [44] . The native-PAGE results indicated that a large-sized complex could be formed by TRPA1a and TRPA1b compared with that of TRPA1a and TRPA1b homo-tetramers. According to the apparent band size of the complex, the complex might be formed in a 1:1 ratio of TRPA1a and TRPA1b, namely four TRPA1a subunits and four TRPA1b subunits. Whole-cell patch-clamp recording data are consistent with the biochemical data in that co-expression of TRPA1a with TRPA1b enhanced TRPA1 activity regardless of activation mechanism, proving functional interaction between TRPA1a and TRPA1b. Surprisingly, single-channel unitary conductance and the open-time kinetics of the complex remained the same as that of TRPA1a homo-tetramer, which indicates that a heteromer of TRPA1a with TRPA1b is less possible. Besides the increased expression level and channel activity of TRPA1a upon co-expression with TRPA1b in HEK293T cells, we also demonstrated that overexpression of TRPA1b in primary DRG neurons increased AITC-, but not capsaicin-evoked [Ca 2+ ] i responses. Those results indicated that TRPA1b selectively interacted with and regulated TRPA1a, but not TRPV1 in sensory neurons, although there are several reports regarding functional and/or physical interaction between TRPV1 and TRPA1 (ref. 45 ). These results indicated that TRPA1b regulated TRPA1a activity not only in a heterologous expression system but also in native sensory neurons by a mechanism that increased plasma membrane TRPA1a expression level. Even though TRPA1b interacts with and regulates TRPA1a, the relatively low expression level of Trpa1b mRNA compared with Trpa1a under physiological conditions could restrict its physiological significance. However, it is possible that mRNA expression patterns and levels of Trpa1a or Trpa1b could be changed under certain pathological conditions. Indeed, analysis of two well-established mouse pain models (CFA-induced inflammatory pain and PSL-induced neuropathic pain models) confirmed this hypothesis. Both expression patterns of Trpa1a and Trpa1b mRNAs changed dynamically in these models. Similar to the previous studies [8] , [33] , Trpa1a mRNA increased in the early stage of inflammatory pain and returned to the basal level. In contrast, the Trpa1b mRNA level increased slowly for 2 weeks after CFA injection or PSL operation. The fact that the response of TRPA1a to AITC was enhanced when TRPA1a and TRPA1b were co-expressed at a ratio of 2:1 suggests that a small increase in TRPA1b in pathological conditions possibly enhances TRPA1a expression, leading to the increased TRPA1 activity. These interesting results could explain how TRPA1 expression contributed to mechanical hyperalgesia with such rapid rates of increase and decrease. According to our study, increased Trpa1a expression in the early inflammation stage is sufficient to contribute to mechanical hyperalgesia, but in later stages when Trpa1a expression has returned to basal level, the slowly but significantly increased amount of Trpa1b could maintain TRPA1a expression at a level that could sustain mechanical hyperalgesia. Similar to the inflammatory pain model, we observed a rapid and transient increase in Trpa1a expression and slow and sustained increase in Trpa1b in the PSL-induced neuropathic pain model. This sustained increase in Trpa1b could be involved in the prolonged mechanical hyperalgesia in the neuropathic pain model as also observed in the inflammatory pain model. Alternative splicing is a well-characterized enzyme-mediated process that is precisely regulated by several critical proteins [46] . Interestingly, recent studies indicated that there is a relationship between different kinds of diseases and alternative splicing [47] , [48] . The best-studied splice regulators are members of the SR (serine and arginine) proteins and hnRNP families. If the enzymatic activities of these proteins were affected during some pathologic states, such as inflammation, it is easy to imagine that alternative splicing would also be changed and diversify the products from the pre-mRNAs. However, the mechanistic relationships between various kinds of diseases and alternative splicing remain largely unknown. Recently, much progress has been achieved concerning the relationship between inflammatory disease and alternative splicing. Inflammatory factors, such as cytokines, are believed to be capable of altering pre-mRNA alternative splicing in pancreatic β-cells [49] . Similar relationships have also been described in many other reports [48] , [50] , [51] . The relation between changes in Trpa1b and inflammation could be explained in a similar way although the precise mechanisms for the dynamic changes in Trpa1a and Trpa1b expression patterns remain unclear. In summary, this study has identified a mouse TRPA1 alternative splice variant, TRPA1b, which interacts with TRPA1a. Furthermore, dynamic changes are observed in Trpa1a and Trpa1b expression patterns under CFA-induced inflammatory and PSL-induced neuropathic pain conditions. These results could provide new insights for understanding the relationship between diseases and alternative splicing of ion channels. Animals Male C57Bl/6NCr mice (4–6-week old) and SD rats (3-week old) were housed in a controlled environment (12 h light/dark cycle; 25 °C; 50–60% humidity) with food and water ad libitum . For the inflammatory pain model, 20 μl CFA was administered to the left hind paw. For the neuropathic pain model, the mice were anesthetized and the right sciatic nerve was exposed. Part of the sciatic nerve was transected with a thread. Saline-injected and sham-operated mice served as controls. The 50% mechanical thresholds were determined with a von Frey test by an up–down method of Dixon [52] on days 1, 2, 5, 7 and 14. The mice were killed after 1, 5, 7 and 14 days for qRT–PCR, and for calcium-imaging experiments after 14 days. All procedures involving the care and use of animals were approved by the Institutional Animal Care and Use Committee of the National Institutes of Natural Sciences and carried out in accordance with the National Institutes of Health Guide for the care and use of laboratory animals (NIH publication No. 85-23, revised 1985). TRPA1 knockout mice were generously provided by Dr David Julius (UCSF, San Francisco, California, USA). Molecular cloning of TRPA1a and TRPA1b Trpa1a and Trpa1b were cloned into the pcDNA3.1 vector using KOD FX DNA polymerase. Forward and reverse primers were 5′-AAGGATCCGCCACCATGAAGCGCGGC-3′ and 5′-GAGCGGCCGCCTAAAAGTCCGGGTGG-3′ respectively. For tagged vector construction, forward and reverse primers were 5′-AAGCTAGCGCCACCATGAAGCGCGGC-3′ and 5′-AAGGTACCGCAAAGTCCGGGTGG-3′ for Trpa1a , 5′-AAGGATCCGCCACCATGAAGCGCGGC-3′ and 5′-AAGCGGCCGCAAAGTCCGGGTGG-3′ for Trpa1b . After Trpa1a was digested with Nhe I and Kpn I and Trpa1b with Bam HI and Not I, they were subcloned into pEGFP-N1 and pcDNA-FLAG vectors, respectively. RT–PCR and single-cell RT–PCR C57Bl/6NCr mouse and SD rat DRG were rapidly collected and total RNA was isolated. Human DRG total RNA was purchased from Clontech Laboratories Incorporation. RT–PCR was performed using the SuperScript III kit from Life Technologies. For single-cell RT–PCR, a glass pipette was used to aspirate cytosolic components from DRG neurons after making a whole-cell configuration. RT–PCR was performed in the same way as above. RT–PCR products were purified by ethanol precipitation and the pellets were used for the second PCR by using the same primers. Forward and reverse primers were 5′-AACTCCTCAACCACCCTGTG-3′ and 5′-CTGAGGCCAAAAGCCAGTAG-3′ for mouse Trpa1 , 5′-AACTCCACCCCACACTGAAG-3′ and 5′-TCGCCTCTGCAGGAAATACT-3′ for mouse Trpv1 , 5′-GAGCTCCTCAACCACCCTGTG-3′ and 5′-GCTGAGGCCAAAAGCCAATAG-3′ for rat Trpa1 , 5′-GAGCTTCTCAATCATCCTGTG-3′ and 5′-GCTGAGTCCAAAAGCCAGAAGA-3′ for human TRPA1 , 5′-TGTTACCAACTGGGACGACA-3′ and 5′-AAGGAAGGCTGGAAAAGAGC-3′ for β-actin. qRT–PCR Trpa1a and Trpa1b mRNA copy numbers were determined by SYBR Green. Forward and reverse primers were 5′-CAAGTATATTTGGATATTGCAAAGAAG-3′ and 5′-CTGAGGCCAAAAGCCAGTAG-3′ for Trpa1a , 5′-GAATAGACACTCTGAAAAGGAATTAC-3′ and 5′-CTGAGGCCAAAAGCCAGTAG-3′ for Trpa1b , 5′-GACAGGATGCAGAAGGA-3′ and 5′-TGATCCACATCTGCTGGAA-3′ for β-actin. Data were analysed using ABI-7700 SDS software. Maintenance of HEK293T cells and immunocytochemistry Human embryonic kidney-derived 293T (HEK293T) cells were maintained in DMEM containing 10% heat-inactivated FBS, 100 units ml −1 penicillin and streptomycin and 2 mM L -glutamine at 37 °C and 5% CO 2 . HEK293T cells were transfected with the appropriate plasmids using Lipofectamine reagent from Life Technologies. TRPA1a alone group was transfected with 0.1 μg Trpa1a and 0.9 μg empty pcDNA3.1 plasmid. TRPA1b alone group was transfected with 0.9 μg Trpa1b and 0.1 μg empty pcDNA3.1 plasmid. TRPA1a+TRPA1b group was transfected with 0.1 μg Trpa1a and 0.9 μg Trpa1b . After incubation for 18 h, cells were washed two times with PBS and fixed using 4% PFA. Cells were then washed twice with PBS and once with PBS-T, and blocked for 1 h at room temperature. Cells were incubated with an anti-FLAG antibody (Sigma-Aldrich) diluted 1:1,000, for 1 h at room temperature followed by three washes with PBS-T. Anti-mouse Alexa Fluor Dyes 594 (Molecular Probes) was incubated with cells for 1 h at room temperature. After three washes with PBS and three washes with MilliQ water, cells were mounted onto glass slides. Co-immunoprecipitation of TRPA1a and TRPA1b HEK293T cells were transfected using the same transfection ratio and protocol as in the immunocytochemistry experiment. Cells were lysed in 100 μl RIPA lysis buffer with protease inhibitor cocktail. Cell lysates were pre-cleared with protein G Sepharose beads with rotation at 4 °C for 1 h. The supernatants were collected after centrifugation and incubated with 1 μl anti-FLAG (Sigma-Aldrich) or 1 μl anti-EGFP (Wako Pure Chemical Industries) antibody overnight at 4 °C. Samples were precipitated with 20 μl protein G Sepharose beads for 1 h. Samples were denatured at 95 °C for 5 min, separated on a 6% SDS–PAGE gel and transferred onto a PVDF membrane. The membrane was blocked overnight at 4 °C and then incubated with an anti-EGFP antibody or anti-FLAG antibody, each diluted 1:1,000, for 1 h at room temperature. After three washes with PBS-T, the membrane was incubated for 1 h at room temperature with an anti-mouse IgG HRP-linked antibody (Cell Signaling Technology) diluted 1:5,000. DRG immunoprecipitation DRG cells were rapidly isolated from 10 mice and lysed in 500 μl RIPA buffer with protease inhibitors. Half amount of protein was treated with a deglycosylation enzyme (New England Biolabs) at 37 °C for 4 h. Protein was added to 10 μl rabbit anti-mouse TRPA1 polyclonal antibody (generously provided by Dr Noguchi). Proteins and antibodies were incubated with rotation at 4 °C overnight, then 50 μl Protein G Mag Sepharose (Life Technologies) was added and incubated at 4 °C for 9 h. After incubation, the supernatant was removed and beads were washed twice with TBS buffer. Proteins were eluted by adding SDS with 100 mM DTT at 95 °C for 5 min. Native-PAGE HEK293T cells were transfected with plasmids using the same transfection ratio and protocol as in the immunocytochemistry experiment. HEK293T cells were harvested on ice and lysed in 100 μL RIPA buffer without detergent. Cell lysates were separated on 4–15% Mini-Protean TGX Gels (Bio-Rad) and transferred onto PVDF membranes. The membranes were blocked overnight and incubated with anti-FLAG or anti-EGFP antibodies diluted 1:1,000. After three washes with PBS-T, the membranes were incubated with for 1 h at room temperature with an anti-mouse IgG HRP-linked antibody diluted 1:5,000. Plasma membrane protein biotinylation HEK293T cells were transfected with plasmids using the same transfection ratio and protocol as in the immunocytochemistry experiment. HEK293T cells were washed three times with PBS and incubated twice with 0.5 mg ml −1 EZ-Link NHS-SS-Biotin (Pierce) for 20 min each. Cells were washed three times with quenching buffer (100 mM glycine in PBS, pH 8.0) and twice with PBS. Cells were collected and lysed in RIPA lysis buffer with complete protease inhibitor cocktail. Biotinylated proteins were precipitated overnight using 10 μl Streptavidin–agarose beads with rotation at 4 °C. Beads and eluates were separated by a spin column, and denatured at 95 °C for 5 min with SDS and DTT. Samples were analysed by western blotting. Quantification of western blot bands was performed using Image J software. Full gel images of PCR and western blotting experiments can be found in Supplementary Fig. S2 . DRG isolation and electroporation Mouse DRG cells from L4 and L5 sections were rapidly isolated and enzymatically digested. After digestion, cells were gently dissociated using fire-polished Pasteur pipettes. Cells were then seeded onto poly- D -lysine pre-coated cover slips. Calcium imaging was carried out after incubation overnight. For DRG electroporation, cells were resuspended with 1 ml PBS (−) after dissociation and 10 μg mouse TRPA1b and 1 μg pCMV-DsRed plasmids was electroporated into DRG by the Neon transfection system. Electroporation conditions were as follows: 900 V, 25 ms, two pulses. Calcium imaging was carried out after incubation for 48 h. Calcium imaging and electrophysiology Calcium influx was monitored with 5 μM fura-2 AM. A positive response was obtained when the ratio increases by agonists were more than 0.2. The real cytosolic Ca 2+ concentrations were calculated with a standard curve generated using different concentrations of extracellular Ca 2+ with 5 μM ionomycin [53] . For whole-cell patch-clamp experiments, TRPA1a alone group was transfected with 0.1 μg Trpa1a and 0.9 μg empty pcDNA3.1 plasmids. TRPA1b alone group was transfected with 0.9 μg Trpa1b and 0.1 μg empty pcDNA3.1 plasmids. TRPA1a+TRPA1b group was transfected with 0.1 μg Trpa1a and 0.9 μg Trpa1b plasmids. In the experiment that cells were transfected with different ratios, 0.1 μg Trpa1a was transfected together with different amounts of Trpa1b and the total DNA amounts were brought to 1.1 μg with empty pcDNA3.1 plasmid. The standard bath solution contained 140 mM NaCl, 5 mM KCl, 2 mM MgCl 2 , 2 mM CaCl 2 , 10 mM HEPES and 10 mM glucose, pH 7.4, adjusted with NaOH. The pipette solution contained 140 mM KCl, 5 mM EGTA and 10 mM HEPES, pH 7.4, adjusted with KOH. Data were sampled at 10 kHz and filtered at 5 kHz. The membrane potential was clamped at −60 mV during recording and a voltage ramp from −100 mV to +100 mV in 500 ms was applied for 5 s. For inside-out single-channel patch-clamp, the pipette solution was substituted with standard bath solution, whereas the extracellular solution was changed to pipette solution used in whole-cell recording. Single-channel data were sampled at 10 kHz and filtered at 2 kHz. Data were recorded using pClamp and analysed using Clampfit software. Statistical analysis Group data represent the mean±s.e.m. Statistical analysis was performed with Student’s t -test or one-way ANOVA with Bonferroni’s post hoc analysis. P <0.05 was considered to be significant. Accession codes: The nucleotide sequence for the Trpa1 splice variant reported in this paper has been deposited in GenBank under accession code KF460461 . How to cite this article: Zhou, Y. et al. Identification of a splice variant of mouse TRPA1 that regulates TRPA1 activity. Nat. Commun. 4:2399 doi: 10.1038/ncomms3399 (2013).